Selective synthesis of tightly- and loosely-twisted metallomacrocycle isomers towards precise control of helicity inversion motion 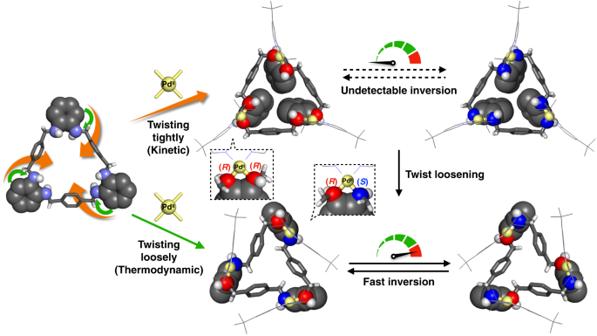Fig. 1: The concept of molecular helicity inversion controlled by twisting mode due to differences in the absolute configurations of the diamine moieties locked by the metal ions. Colour: Pd yellow, C black, H white, N Purple (non-coordinated), red (R-configuration) and blue (S-configuration). Molecular twist is a characteristic component of molecular machines. Selectively synthesising isomers with different modes of twisting and controlling their motion such as helicity inversion is an essential challenge for achieving more advanced molecular systems. Here we report a strategy to control the inversion kinetics: the kinetically selective synthesis of tightly- and loosely-twisted isomers of a trinuclear Pd II -macrocycle and their markedly different molecular behaviours. The loosely-twisted isomers smoothly invert between ( P )- and ( M )-helicity at a rate of 3.31 s –1 , while the helicity inversion of the tightly-twisted isomers is undetectable but rather relaxes to the loosely-twisted isomers. This critical difference between these two isomers is explained by the presence or absence of an absolute configuration inversion of the nitrogen atoms of the macrocyclic amine ligand. Strategies to control the helicity inversion and structural loosening motions by the mode of twisting offer future possibilities for the design of molecular machines. One of ultimate goals in the chemistry of molecular machines is to reproduce motions in the macroscopic world at the level of molecules or their aggregates. A number of excellent examples of molecular machines have been reported to control a variety of motions, including rotation [1] , [2] , [3] , [4] , [5] and translation [6] , [7] , [8] , [9] , [10] . However, controlling motion elements such as directionality [3] , [11] , speed [4] , [10] and frequency (ON/OFF) [9] , [12] is still a major challenge. For example, Stoddart et al. controlled the translational motion of rings shuttling along the axles by redox or acid/base [6] . Feringa et al. reported unidirectional molecular rotors based on photo- and thermal-isomerisation of olefins [11] . In addition to these motions, twisting motion and its inversion motion have recently attracted much attention in terms of motion complexity and asymmetry, leading to advanced molecular machines and chiral memory [13] , [14] , [15] , [16] , [17] . We intuitively understand that the twisting behaviours are highly dependent on the mode of twisting. For instance, a loosely-twisted object will unwind easily, but a very tightly-twisted object may not. Can such movements be reproduced in the nanoscale world? Inspired by biomacromolecules, chemists have synthesised twisted molecules such as helical polymers [18] , [19] , [20] , helicenes [21] , [22] and twisted macrocycles [23] , [24] , [25] , and in some of these examples, the design and control of their twisting motion are being studied. For instance, the rate of helicity inversion was controlled by exploiting the kinetic properties of coordination bonds in twisted metal complexes of synthetic peptides [26] , macrocycles [27] and cryptands [28] . Another role of metal coordination is to dynamically fix the absolute configuration of the coordinating atoms, including the amine nitrogen atoms, which is usually immediately reversed. Thus, selective synthesis of metal complexes with different modes of twisting resulting in different configurations and/or conformation, or twisted isomers is a promising strategy to control the inversion motion without changing the chemical composition, but such isomers are limited to a few examples [29] , [30] , [31] , [32] . Thus, it is still challenging to selectively synthesise such twisted isomers. Molecular motion is described by a combination of rotational and translational motions, but various modes are possible depending on the shape and size of the molecule itself, the flexibility of the structure derived from the bonding modes and the environment surrounding the molecule. Molecular twist is a mode included in many molecular motions of molecular machines. Selective synthesis of isomers with different mode of twisting and control of their motion such as inversion, is an indispensable task to realise more advanced molecular systems. Herein we report the selective synthesis of two twisted isomers of a trinuclear Pd II -macrocycle with a tightly- or loosely-twisted skeleton (Fig. 1 ). It is particularly important to emphasise that these two isomers have markedly different rates of helicity inversion depending on the mode of twisting with different absolute configurations of the diamine moieties locked by the metal ions. The loosely-twisted isomer exhibited rapid helicity inversion, whereas the helicity inversion in the tightly-twisted isomer was actually undetectable because the inversion process requires absolute configuration inversion of the nitrogen atoms. In other words, the helicity inversion of the twisted macrocycle is configurationally inhibited by twisting more tightly. Thus, this result is an excellent example of twisting motion controlled by the mode of twisting of a single chiral molecule with coordinating atoms of different configurations. Fig. 1: The concept of molecular helicity inversion controlled by twisting mode due to differences in the absolute configurations of the diamine moieties locked by the metal ions. Colour: Pd yellow, C black, H white, N Purple (non-coordinated), red ( R -configuration) and blue ( S -configuration). Full size image Selective synthesis of two twisted isomers, 1 tight and 1 loose (Fig. 2 ) Previously, our group synthesised helically-twisted Pd II -macrocycles, [Pd 3 L Cl 6 ], from an achiral macrocyclic hexaamine ligand L and 3 equiv. of [PdCl 2 (CH 3 CN) 2 ] in CH 2 Cl 2 :DMSO = 9/1 (v/v) [33] . The C 3 -symmetric macrocyclic skeleton with three Pd II centres on the same side was helically twisted by intramolecular C-H···π interactions (Fig. 3i, j ). This complex exhibits helicity inversion between the ( P )- and ( M )-enantiomers with an inversion rate of 14 s –1 at 292 K in CD 2 Cl 2 :DMSO- d 6 = 9/1 (v/v). In this study, we aimed to significantly modulate the rate of helicity inversion by replacing all two chloride ligands on the three Pd II centres with 4,4’-di- tert -butyl-2,2’-bipyridine ( t Bu 2 bpy) ligands. First, we attempted to synthesise a twisted Pd II -macrocycle with Pd( t Bu 2 bpy) moieties in a manner similar to our previous study [33] . Ligand L was reacted with 3.2 equiv. of [Pd( t Bu 2 bpy)(OH 2 ) 2 ](OTf) 2 in CH 2 Cl 2 at room temperature for 4 h. After removal of the solvent, the residue was recrystallised to afford colourless crystals 1 tight in 33% yield (Fig. 2 ). The composition was determined by elemental analysis to be [Pd 3 L ( t Bu 2 bpy) 3 ](OTf) 6 ·(H 2 O) 4.9 ·(Et 2 O) 0.15 . Single-crystal X-ray diffraction (ScXRD) analysis revealed that [Pd 3 L ( t Bu 2 bpy) 3 ](OTf) 6 has a C 3 -symmetric twisted structure (Fig. 3a–c ), and the twisting macrocyclic structure was different from that of [Pd 3 L Cl 6 ] (Fig. 3j ). Specifically, the three ortho -phenylenediamine moieties folded inside the macrocycle to form a tightly-twisted skeleton, and this complex [Pd 3 L ( t Bu 2 bpy) 3 ](OTf) 6 is referred to here as the tightly-twisted isomer ( 1 tight ): the other loosely-twisted isomer ( 1 loose ) will be discussed below (the definition of the twisted isomers; see the Supplementary Section 2 . 4 ). This isomer 1 tight has ( P )- or ( M )-helicity, defined by the direction from the para -phenylene rings toward the inner amine protons (Fig. 2 ), and both enantiomers crystallised as a racemate. Unlike [Pd 3 L Cl 6 ], 1 tight had three amine protons facing outward of the macrocycle and the other three facing inward, forming hydrogen bonds with one triflate ion in the cavity. The absolute configurations of the six nitrogen atoms, the chiral centres in the ( P )- and ( M )-enantiomers, were therefore all - R - and all - S -configuration, respectively. Intramolecular C-H···Pd interactions between one of the protons of para -phenylene and the Pd centre were suggested by the H···Pd distance (2.74 Å) and the C-H···Pd angle (120°) as one factor stabilising the tightly-twisted structure. These are consistent with typical anagostic interactions (2.3–2.9 Å, 110–170°) [34] . To confirm the structure in solution, the crystals were then dissolved in acetone or dichloromethane and analysed by 1D 1 H and 19 F NMR spectroscopies, 2D NMR spectroscopies ( 1 H− 1 H COSY and ROESY), and high resolution-electrospray ionization time-of-flight (HR-ESI-TOF) mass spectrometry ( m / z = 1100.2498 as [Pd 3 (H –1 L )( t Bu 2 bpy) 3 (OTf) 3 ] 2+ ) (Supplementary Figs. 4 – 16 ). The 19 F NMR spectrum showed two separate triflate signals, one of which was assigned to a triflate incorporated within the macrocycle (Supplementary Fig. 6 ). Two sets of diastereotopic methylene proton signals (H c–f ) were observed in the 1 H NMR spectrum in acetone- d 6 , indicating that the structure is chiral (Fig. 3a, d ). Notably, the downfield shift of one para -phenylene signal (H l ) to 9.8 ppm even at 300 K suggested the presence of a C-H···Pd interaction (Supplementary Fig. 14 ). Moreover, an ortho -phenylenediamine proton signal (H g ) was highly upfield shifted to 4.9 ppm due to the shielding effect from the adjacent ortho -phenylenediamine moieties clustered inside the macrocycle. These results suggest that the tightly-twisted structure is maintained in solution. The interactions suggested by ScXRD and NMR analyses were well supported by natural bond orbital (NBO) and noncovalent interaction (NCI) plot analyses after optimising the geometry with density functional theory (DFT) calculations (Supplementary Figs. 118 – 120 ). 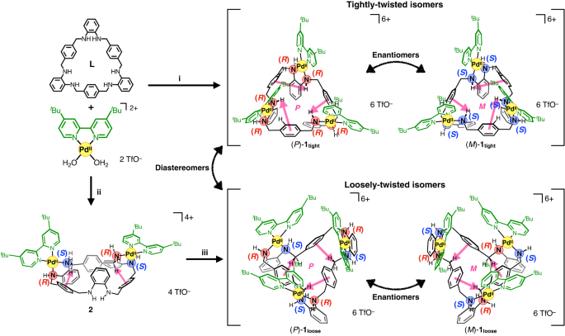Fig. 2: Synthesis of two isomeric PdIIcomplexes, 1tightand 1loose, and the absolute configuration of the amine nitrogen atoms. i CH2Cl2, rt, 4 h, 33%. ii CHCl3, rt, 3 h, 64%. iii [Pd(tBu2bpy)(OH2)2](OTf)2, CH2Cl2, rt for 3 h then reflux for 1.5 h, 49% (31% in two steps). Fig. 2: Synthesis of two isomeric Pd II complexes, 1 tight and 1 loose , and the absolute configuration of the amine nitrogen atoms. i CH 2 Cl 2 , rt, 4 h, 33%. ii CHCl 3 , rt, 3 h, 64%. iii [Pd( t Bu 2 bpy)(OH 2 ) 2 ](OTf) 2 , CH 2 Cl 2 , rt for 3 h then reflux for 1.5 h, 49% (31% in two steps). Full size image Fig. 3: Characterisation of the two twisted isomers of 1. a Substructural formula of 1 tight . b , c Side and top views of the crystal structure of 1 tight with one triflate incorporated via multipoint hydrogen bonding. Hydrogen atoms except amine and methylene moieties are omitted for clarity. d 1 H NMR spectrum (500 MHz, acetone- d 6 , 300 K) of 1 tight . e Substructural formula of 1 loose . f , g Side and top views of the crystal structure of 1 loose with one triflate disordered in the inner space. Hydrogen atoms except amine and methylene moieties are omitted for clarity. h 1 H NMR spectrum (500 MHz, acetone- d 6 , 300 K) of 1 loose . i , j Structural formula and the reported crystal structure (top view) of [Pd 3 L Cl 6 ] [33] . Full size image To synthesise another isomeric trinuclear Pd II -macrocycle with a skeleton similar to [Pd 3 L Cl 6 ], we optimised the reaction conditions and found that a dinuclear Pd II -macrocycle is a key intermediate for the selective synthesis of the other isomers (Fig. 2 ). When ligand L was reacted with 1.6 equiv. of [Pd( t Bu 2 bpy)(OH 2 ) 2 ](OTf) 2 in CHCl 3 at room temperature, a dinuclear [Pd 2 L ( t Bu 2 bpy) 2 ](OTf) 4 ( 2 ) complex precipitated. Its meso -twisted skeleton with two intramolecular C-H···π interactions was deduced from the crystal structure of a Pt II -analogue, 1D and 2D NMR and HR-ESI-TOF mass analyses ( m / z = 689.2654 as [Pd 2 (H –2 L )( t Bu 2 bpy) 2 ] 2+ ) (Supplementary Figs. 34 – 45 ). Dinuclear complex 2 was then reacted again with 1.2 equiv. of [Pd( t Bu 2 bpy)(OH 2 ) 2 ](OTf) 2 in CH 2 Cl 2 , and the product was recrystallised to afford colourless crystals 1 loose , [Pd 3 L ( t Bu 2 bpy) 3 ](OTf) 6 ·(H 2 O) 4 , in 31% total yield. ScXRD analysis revealed that the crystals were composed of another C 3 -symmetric trinuclear complex with a twisted skeleton similar to [Pd 3 L Cl 6 ] (Fig. 3e–g, i, j ). Unlike 1 tight , the three ortho -phenylenediamine moieties were not folded much and located outside the macrocyclic structure, instead, the inside was filled with para -phenylene and three methylene moieties, forming C-H···π interactions between them. Thus, this complex [Pd 3 L ( t Bu 2 bpy) 3 ](OTf) 6 ( 1 loose ) can be regarded as a loosely-twisted isomer of 1 tight . This isomeric complex also formed racemic crystals consisting of ( P )- and ( M )-enantiomers. In contrast to 1 tight , all six amine protons of 1 loose were located outside of the macrocyclic structure, resulting in an alternating R - and S -absolute configuration of nitrogen atoms. Therefore, helicity inversion between the ( P )- and ( M )- 1 loose preserves the alternate absolute configurations ( alt - R / S ) of the nitrogen atoms. One triflate ion was found to be disordered in the space surrounded by three bipyridine portions. Analyses of 1 loose dissolved in acetone by 1D and 2D NMR spectroscopies and HR-ESI-TOF mass spectrometry ( m / z = 1100.2410 as [Pd 3 (H –1 L )( t Bu 2 bpy) 3 (OTf) 3 ] 2+ ) revealed that the structure of 1 loose in solution is consistent with the crystal structure (Supplementary Figs. 19 – 29 ). For instance, one methylene signal (H c ) was upfield shifted to 1.9 ppm in 1 H NMR, which supported the C-H···π interactions observed in the crystal structure (Fig. 3f, g ). This interaction was also supported by NBO and NCI plot analyses after geometry optimisation using DFT calculation (Supplementary Figs. 126 and 127 ). 1 loose was stable in acetone- d 6 at room temperature for two weeks, as evidenced by 1 H NMR analysis (Supplementary Fig. 32 ). In contrast, 1 tight was less stable and slowly isomerised to 1 loose in acetone -d 6 while also producing non-assignable by-products. The isomerisation rate of 1 tight to 1 loose in acetone- d 6 at 293 K was estimated to be (5.7 ± 0.4) × 10 –6 s –1 by the time course 1 H NMR analysis, assuming the isomerisation to be a pseudo first order reaction (Supplementary Section 3 ). This result indicates that 1 tight and 1 loose are the kinetic and thermodynamic products in acetone, respectively, and is consistent with the fact that 1 tight is obtained kinetically under mild conditions in CH 2 Cl 2 . As mentioned above, dinuclear complex 2 , which preferentially precipitated when reacted with less than 2 equiv. of Pd II salts in CHCl 3 , is an important intermediate for the selective synthesis of 1 loose . This result is consistent with the fact that the absolute configuration of the four Pd II -coordinated amine nitrogen atoms in 2 is the same as that of 1 loose and no configurational change is required when 2 is converted to 1 loose . In contrast, to convert to 1 tight with an all - R - or all - S -configuration, 2 requires a configurational inversion of the two Pd II -coordinated amine nitrogen atoms. Thus, the conversion from 2 to 1 tight is kinetically undesirable, resulting in a selective conversion to 1 loose (Fig. 2 ). The difference in the absolute configuration of the Pd II -coordinated amine nitrogen atoms is thus a notable structural difference between 1 tight and 1 loose . It is noteworthy that the two diastereomers can also be regarded as in / out -isomers if we focus on the nitrogen-containing cyclic structures, which is usually applied to bridged bicyclic compounds [35] . Here, the two nitrogen atoms of one ortho -phenylenediamine moiety are the bridgehead atoms of the bicyclic structure bridged via Pd II . According to the definition of in / out -isomers, 1 tight and 1 loose correspond to the in , out - and out , out -isomers, respectively, from the direction of the N-H moieties. Estimation of helicity inversion rate by exchange spectroscopy (EXSY) The inversion rates of 1 loose and 1 tight were then investigated. The helicity inversion rate ( k ) between ( P )- and ( M )- 1 loose was evaluated using EXSY with varying mixing time. The rate constant ( k ) was calculated using the ratio of integrations of chemical exchange signals (e.g., H o and H v for different bipyridine moieties) produced by helicity inversion, which was 3.31 ± 0.02 s –1 at 300 K in acetone- d 6 (Fig. 4a–c , Supplementary Sections 4 . 1 , 4 . 3 ). In the EXSY analysis, the rate constant ( k ) obtained was defined as the sum of the rate constants of the helicity inversion from ( P )- to ( M )- 1 loose ( k PM ) and from ( M )- to ( P )- 1 loose ( k MP ) (Fig. 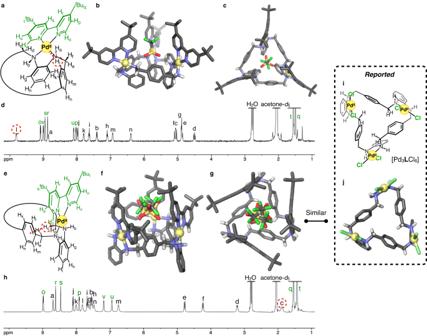Fig. 3: Characterisation of the two twisted isomers of 1. aSubstructural formula of1tight.b,cSide and top views of the crystal structure of1tightwith one triflate incorporated via multipoint hydrogen bonding. Hydrogen atoms except amine and methylene moieties are omitted for clarity.d1H NMR spectrum (500 MHz, acetone-d6, 300 K) of1tight.eSubstructural formula of1loose.f,gSide and top views of the crystal structure of1loosewith one triflate disordered in the inner space. Hydrogen atoms except amine and methylene moieties are omitted for clarity.h1H NMR spectrum (500 MHz, acetone-d6, 300 K) of1loose.i,jStructural formula and the reported crystal structure (top view) of [Pd3LCl6]33. 4a ) [36] . The Gibbs free energy (Δ G ‡ ), enthalpy (Δ H ‡ ) and entropy (Δ S ‡ ) of activation at 300 K were estimated to be 70.6 ± 1.3 kJ/mol, 86.1 ± 0.9 kJ/mol and 51.9 ± 3.1 J/(mol·K), respectively, by the Eyring plot based on the inversion rate at temperatures varying in the range from 280 to 310 K (Supplementary Figs. 50 – 52 ). The large positive entropy of activation is probably due to the formation of lower symmetry structures in the transition state and the release of anions and solvent molecules. The inversion rate obtained here is nearly equivalent to that of [Pd 3 L Cl 6 ] with a loosely-twisted conformation ( k = 14 s –1 at 292 K in CD 2 Cl 2 /DMSO- d 6 ) [33] , although the ligands and conditions are different. The relatively fast inversion rate of the loosely-twisted complexes is consistent with the argument, discussed earlier, that the helicity inversion does not require configurational inversion of the amine nitrogen atoms. Fig. 4: Estimation of the helicity inversion rate. a Scheme of the helicity inversion between ( P )- and ( M )- 1 loose . b EXSY spectrum (500 MHz, acetone- d 6 , 300 K, mixing time = 0.3 s, 0.19 mM) of ( P / M )- 1 loose . The chemical exchange signals between H o and H v ( ex o-v), flamed in blue, were used to estimate the inversion rate. c Partial structural formula of 1 loose . d Scheme of the helicity inversion between ( P )- and ( M )- 1 tight . e EXSY spectrum (500 MHz, acetone- d 6 , 300 K, mixing time = 0.3 s) of ( P )- and ( M )- 1 tight . No chemical exchange signals between H o and H v were observed, as shown in the blue dotted boxes. f Partial structural formula of 1 tight . Full size image In contrast, no chemical exchange signals between H o and H v were observed in the EXSY spectra of 1 tight in acetone- d 6 at 300 K (Fig. 4d–f ). This suggests that the inversion rate of 1 tight is too slow to be evaluated by EXSY. Compared to 1 loose , the helicity inversion of 1 tight requires configurational inversion of all amine nitrogen atoms, as described above, which slows the inversion rate. The triflate incorporated into the interior of the macrocycle may also contribute to stabilising the absolute configuration of the inward amine nitrogen atoms via hydrogen bonding. Therefore, we next attempted to synthesise enantio-enriched 1 tight using a chiral auxiliary and estimated its racemisation rate as the helicity inversion rate. Asymmetric synthesis of 1 tight Asymmetric synthesis of enantio-enriched 1 tight was investigated using chiral sulfoxides as additives (Fig. 5 ). Among several chiral sulfoxides examined, ( R / S )-mesityl methyl sulfoxide (( R / S )- 3 ) was the best in terms of product yield and optical purity (Fig. 5c, d and Supplementary Fig. 96 ). Specifically, 3.2 equiv. of [Pd( t Bu 2 bpy)(OH 2 ) 2 ](OTf) 2 was mixed with an excess of ( S )- 3 and reacted with L in CH 2 Cl 2 at –70 °C for 4 h (Fig. 5a ). After washing ( S )- 3 , enantio-enriched 1 tight was obtained in 15% yield. The enantiomeric excess of the product was determined to be 25% ee by 1 H NMR in CD 2 Cl 2 containing Δ-TRISPHAT tetrabutylammonium salt (Δ- 4 ) as a chiral shift reagent (Fig. 5e, f and Supplementary Fig. 90 ). Δ- 4 had no effect on the enantiomeric ratios of the products, as evidenced by time-course 1 H NMR analysis of racemic and enantio-enriched 1 tight (Supplementary Figs. 114 – 117 ). The product was pure enough for further analysis and was not recrystallised to prevent changes in enantiomeric excess. When analysed by circular dichroism (CD) spectroscopy, this product exhibited a negative Cotton effect at 325 nm in CH 2 Cl 2 (Fig. 5b (red line)). Using enantiomer ( R )- 3 , the other enantio-enriched 1 tight with opposite chirality was synthesised in the same way, and the product showed a positive Cotton effect at 325 nm in the CD spectrum (Fig. 5b (blue line)). The mirror image of the CD spectra indicated that the asymmetric synthesis was successfully achieved by chiral 3 . Fig. 5: Asymmetric synthesis of 1 tight . a Synthesis of ( M )-enantio-enriched 1 tight . b CD spectra (CH 2 Cl 2 , 293 K, l = 1.0 cm) of ( P )- and ( M )-enantio-enriched 1 tight (blue and red lines, respectively). Structural formula of ( R )- 3 c , ( S )- 3 d and Δ-TRISPHAT tetrabutylammonium salt (Δ- 4 ) e . f Partial 1 H NMR spectra (500 MHz, CD 2 Cl 2 , 300 K) of the ( M )-enantio-enriched 1 tight with Δ- 4 . The upper spectrum (day 0) was recorded by dissolving the as-synthesised product in CD 2 Cl 2 containing Δ- 4 . The lower spectrum (day 3) was obtained by dissolving the product in acetone- d 6 , allowing it to stand at 293 K for 3 days, evaporating the solution at room temperature and then redissolving in CD 2 Cl 2 containing Δ- 4 . Day 0 and day 3 enantiomer excesses were evaluated by the integral of the signals after deconvolution. g 1 H NMR analysis (500 MHz, acetone- d 6 , 300 K) of the ( M )-enantio-enriched 1 tight without Δ- 4 dissolved in acetone- d 6 after 0 day (upper) and 3 days (lower). Signals of 1 loose are indicated by orange triangles. Full size image Time dependent-DFT calculations [M06-D3/def2svp for Pd, 6-31G(d) for other atoms] were then performed to determine the absolute structures of both enantio-enriched 1 tight . The calculated CD spectrum of the optimised ( P )- 1 tight qualitatively reproduced the experimental spectrum of the enantio-enriched 1 tight synthesised with ( R )- 3 (Supplementary Fig. 121 ). For example, positive Cotton effects in the low energy region were found in both the experimental and calculated spectra. Similar results were obtained in the calculations of CD spectra with other functionals or basis sets (Supplementary Figs. 122 – 125 ). These support that the ( P )- and ( M )-enantio-enriched 1 tight were synthesised with ( R )- and ( S )- 3 , respectively. Helicity inversion versus twist loosening observed in 1 tight (Fig. 6 ) The helicity inversion rate was evaluated using ( M )-enantio-enriched 1 tight . An acetone- d 6 solution of the ( M )-enantio-enriched 1 tight ( P : M = 37:63) was allowed to stand at 293 K for 3 days (Fig. 5g ). After the solvent was removed, the enantiomeric ratio was examined using Δ- 4 in CD 2 Cl 2 , and its enantiomeric ratio ( P : M = 38:62) was almost the same as that of the starting material. This indicates that either the helicity inversion is too slow to be detected or that the inversion of 1 tight does not occur under this condition (Fig. 5f , Supplementary Sections 7.1 – 7.2 ). Similarly, the inversion rate in CD 2 Cl 2 was also examined at 293 K, but no inversion was observed in 10 days (Supplementary Figs. 112 and 113 ). Besides, 1 tight gradually isomerised to 1 loose as described above, and the isomerisation to 1 loose was observed during these analyses. These results suggest that the rate of isomerisation from 1 tight to 1 loose (twist loosening) (5.7 × 10 –6 s –1 ) is faster than that between ( P )- and ( M )- 1 tight (helicity inversion). The faster isomerisation from 1 tight to 1 loose can be explained from the number of amine nitrogen atoms whose absolute configuration inverts. That is, in the case of ( all - R ) or ( all - S ) → ( alt - R / S ) (twist loosening), only three of the six amine portions need to be inverted, but in the case of ( all - R ) ⇄ ( all - S ) (helicity inversion), all six amine portions must be inverted. Since configurational inversion of the amine moieties involves dissociation of the N–Pd or N–H bonds, the number of nitrogen inversion sites may affect the isomerisation rate. This consideration is also applied to understanding that the helicity inversion of 1 loose (1.38 s –1 at 293 K, estimated by the Eyring plot, Supplementary Fig. 52 ) is much faster than that of 1 tight . This is because the helicity inversion of 1 loose does not require the configurational changes of amine nitrogen atoms (( alt-R/S ) ⇄ ( alt-R/S )). On the other hand, the inversion of the all - R or all - S configuration in 1 tight probably needs to occur in a stepwise manner via the intermediary alt - R / S configuration, but the intermediate corresponding to thermodynamically stable 1 loose is no longer isomerised to the all - S or all - R configuration, respectively (Fig. 7 ). Fig. 6: Helicity inversion versus twist loosening of 1 tight . Undetectable helicity inversion between ( P )- and ( M )- 1 tight , twist loosening from 1 tight to 1 loose and fast helicity inversion between ( P )- and ( M )- 1 loose . Full size image Fig. 7: Possible isomers and their isomerisation pathways of 1. All possible diastereomers and their isomerisation pathways for 1 are shown in this scheme. The black circles indicate the helically twisted macrocyclic structures of 1 . The notions RR , SS and SR above the black circles indicate pairs of the absolute configurations of the amine nitrogen atoms of the ortho -phenylenediamine moiety observed in the crystal strictures. The isomerisation pathways to the RS configuration are excluded in this scheme, as a pair of the amine nitrogen atoms with the RS configurations, with the two amine protons pointing towards the inside of the macrocycle, was not observed experimentally. The green arrows indicate the direct isomerisation pathways from 1 tight to 1 loose , and the dotted arrows indicate other possible isomerisation pathways. Full size image Finally, 1 tight was found to be more stabilised when the solvent was substituted from acetone- d 6 to CD 2 Cl 2 . The stability of ( M )-enantio-enriched 1 tight was examined by 1 H NMR spectroscopy and it was found that in acetone- d 6 twist loosening and degradation began within 1 day at 293 K, whereas in CD 2 Cl 2 such changes were significantly slower even after 6 days (Supplementary Figs. 109 and 112 ). Of note, the addition of Δ- 4 in CD 2 Cl 2 also markedly inhibited the tight-to-loose isomerisation. 1 H NMR spectra of ( M )-enantio-enriched 1 tight in the presence of Δ- 4 (17 equiv.) showed that most of 1 tight remained without significant isomerisation or degradation at 293 K in CD 2 Cl 2 even after 14 days (Supplementary Fig. 116 ). One possibility is that the Δ-TRISPHAT anion associates with the cationic 1 tight with a similar symmetry to increase the stability, which was supported by the shift and splitting of the 1 H NMR and 19 F NMR signals of the encapsulated triflate (Supplementary Figs. 89 and 115 ). Thus, a very slow or no inversion can be switched to a faster inversion by isomerisation from a tight to a loose state, and the switching speed can be adjusted by additives or solvents. In this study, we have succeeded in selectively synthesising two twisted isomers of trinuclear Pd II -macrocycles with markedly different rates of helicity inversion. In the tightly-twisted isomer 1 tight , the three ortho -phenylenediamine moieties were folded inside the macrocyclic skeleton and the absolute configurations of the amine nitrogen atoms were all - R or all - S , while in the loosely-twisted isomers 1 loose , the three ortho -phenylenediamine moieties were folded outside the skeleton and the absolute configurations of the amine nitrogen atoms were alt - R / S . In stark contrast to 1 tight , which shows a very slow or no inversion, 1 loose exhibits fast helicity inversion (1.38 s –1 at 293 K in acetone- d 6 ). Moreover, the inversion kinetics can be controlled by isomerisation in a range from 1 tight , where no inversion is detected, to 1 loose , where inversion is fast. Our approach to the control of helicity inversion motion by the twisted isomers resulting from the configurational locking with metal ions is quite different from conventional approaches that require chemical substitutions or additives to control twisting motions. The new strategy of controlling molecular motions by the mode of twisting with coordinating atoms of different configuration is expected to be applicable to a variety of systems and can be expanded to the design of more sophisticated molecular machines. Synthesis of 1 tight A CH 2 Cl 2 solution (1.0 mL) of L (10.0 mg, 15.9 µmol, 1.0 equiv.) was mixed with a CH 2 Cl 2 solution (2.0 mL) of [Pd( t Bu 2 bpy)(OH 2 ) 2 ](OTf) 2 ·(H 2 O) 2 (38.2 mg, 51.3 µmol, 3.2 equiv. ), and then stirred at room temperature for 4 h. During the reaction, the colour of the solution was changed from pale yellow to purple in a few minutes. The reaction mixture was filtered to remove the precipitate and the filtrate was evaporated. The resulting solid was washed with CHCl 3 and the residue was dried up under reduced pressure. The solid was recrystallised from CH 2 Cl 2 by vapour diffusion of Et 2 O. The obtained plate crystals were washed with a small amount of CHCl 3 and dried up under reduced pressure to afford tightly-twisted 1 tight , [Pd 3 L ( t Bu 2 bpy) 3 ](OTf) 6 ·(H 2 O) 4.9 ·(Et 2 O) 0.15 , (14.3 mg, 5.19 µmol, 33% yield) as a colourless solid. Mp: > 257 °C (decomp.). 1 H NMR (500 MHz, acetone- d 6 , 300 K): δ 9.81 (d, J = 7.0 Hz, 3H), 9.09 (d, J = 6.0 Hz, 3H), 9.00 (d, J = 6.0 Hz, 3H), 8.95 (d, J = 1.5 Hz, 3H), 8.88 (d, J = 2.0 Hz, 3H), 8.85 (d, J = 3.5 Hz, 3H), 8.10 (dd, J = 5.0, 1.0 Hz, 3H), 8.03 (dd, J = 6.0, 1.5 Hz, 3H), 7.98 (d, J = 8.5 Hz, 3H), 7.80 (d, J = 5.5 Hz, 3H), 7.64 (t, J = 8.0 Hz, 3H), 7.41 (d, J = 10.5 Hz, 3H), 7.10 (t, J = 7.5 Hz, 3H), 6.94 (d, J = 7.0 Hz, 3H), 6.40 (d, J = 7.0 Hz, 3H), 5.09 (d, J = 14.5 Hz, 3H), 5.05 (d, J = 15.0 Hz, 3H), 4.89 (d, J = 7.5 Hz, 3H), 4.87 (d, J = 13.5 Hz, 3H), 4.50 (dd, J = 14.0, 11.5 Hz, 3H), 1.56 (s, 27H), 1.50 (s, 27H). 13 C NMR (126 MHz, acetone- d 6 , 301 K): δ 168.9, 168.7, 157.8, 157.3, 152.2, 150.4, 142.0, 141.8, 134.5, 134.2, 133.4, 133.1, 132.1, 131.9, 131.2, 129.2, 128.6, 126.9, 126.6, 126.5, 123.3, 123.2, 122.9, 120.8, 118.2, 63.0, 61.3, 37.1, 37.0. The 13 C signals of tert -butyl groups were overlapped with those of acetone- d 6 and could not be identified. The TfO anion has four 13 C signals but only three signals were observed due to the low S/N ratio. 19 F NMR (471 MHz, acetone- d 6 , 300 K): δ –75.4, –76.1. IR (ATR, cm –1 ): 3144 (br), 2967, 1618, 1417, 1248, 1155, 1028, 810, 636. UV-vis (CH 2 Cl 2 , 293 K, 87.3 µM): λ max (nm) ( ε (M –1 cm –1 )) = 309.8 (3.98 × 10 4 ). HRMS (ESI-TOF): m / z = 1100.2498 as [Pd 3 (H –2 L )( t Bu 2 bpy) 3 ](OTf) 3 ] + (calcd 1100.2462). Anal. 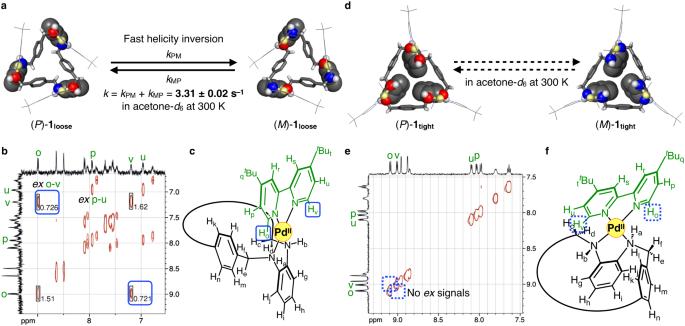Fig. 4: Estimation of the helicity inversion rate. aScheme of the helicity inversion between (P)- and (M)-1loose.bEXSY spectrum (500 MHz, acetone-d6, 300 K, mixing time = 0.3 s, 0.19 mM) of (P/M)-1loose. The chemical exchange signals between Hoand Hv(exo-v), flamed in blue, were used to estimate the inversion rate.cPartial structural formula of1loose.dScheme of the helicity inversion between (P)- and (M)-1tight.eEXSY spectrum (500 MHz, acetone-d6, 300 K, mixing time = 0.3 s) of (P)- and (M)-1tight. No chemical exchange signals between Hoand Hvwere observed, as shown in the blue dotted boxes.fPartial structural formula of1tight. Calcd for C 102.6 H 125.3 F 18 N 12 O 23.05 Pd 3 S 6 {[Pd 3 L ( t Bu 2 bpy) 3 ](OTf) 6 ·(H 2 O) 4.9 ·(Et 2 O) 0.15 }: C 44.82, H 4.58, N 6.09; found: C 44.81, H 4.58, N 6.09. Crystal data for tightly-twisted Pd 3 L ( t Bu 2 bpy) 3 ·(OTf) 5.08 ·(H 2 O) 6.95 ·(CH 2 Cl 2 ) 1.27 (missing triflates were not observed due to severe disorder): C 102.36 H 116.55 Cl 2.55 F 15.25 N 12 O 22.20 Pd 3 S 5.08 , F w = 2732.41, crystal dimensions 0.131 × 0.081 × 0.031 mm 3 , trigonal, space group R -3, a = 23.0889(2), c = 41.6772(6) Å, V = 19241.3(4) Å 3 , Z = 6, ρ calcd = 1.415 g cm –3 , μ = 53.78 cm –1 , T = 93 K, λ (CuK α ) = 1.54187 Å, 2 θ max = 144.478°, 39889/8311 reflections collected/unique ( R int = 0.0578), R 1 = 0.0845 ( I > 2σ( I )), wR 2 = 0.2630 (for all data), GOF = 1.113, largest diff. peak and hole 1.414/–1.123 eÅ –3 . CCDC deposit number 2190130. Synthesis of 1 loose A CHCl 3 solution (2.2 mL) of L (13.2 mg, 20.9 µmol, 1.0 equiv.) was mixed with a CHCl 3 solution (4.7 mL) of [Pd( t Bu 2 bpy)(OH 2 ) 2 ](OTf) 2 ·(H 2 O) 2 (25.2 mg, 33.8 µmol, 1.6 equiv. ), and then stirred at room temperature for 3 h. During the reaction, a pink solid was precipitated. The resulting precipitate was collected by filtration and washed with CHCl 3 to obtain a dark pink solid whose main component was dinuclear metallocycle 2 (21.3 mg, 10.7 µmol, 64%), which was then suspended in CH 2 Cl 2 (10 mL). 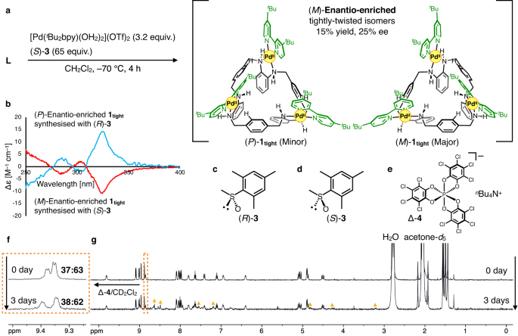Fig. 5: Asymmetric synthesis of 1tight. aSynthesis of (M)-enantio-enriched1tight.bCD spectra (CH2Cl2, 293 K,l= 1.0 cm) of (P)- and (M)-enantio-enriched1tight(blue and red lines, respectively). Structural formula of (R)-3c, (S)-3dand Δ-TRISPHAT tetrabutylammonium salt (Δ-4)e.fPartial1H NMR spectra (500 MHz, CD2Cl2, 300 K) of the (M)-enantio-enriched1tightwith Δ-4. The upper spectrum (day 0) was recorded by dissolving the as-synthesised product in CD2Cl2containing Δ-4. The lower spectrum (day 3) was obtained by dissolving the product in acetone-d6, allowing it to stand at 293 K for 3 days, evaporating the solution at room temperature and then redissolving in CD2Cl2containing Δ-4. Day 0 and day 3 enantiomer excesses were evaluated by the integral of the signals after deconvolution.g1H NMR analysis (500 MHz, acetone-d6, 300 K) of the (M)-enantio-enriched1tightwithout Δ-4dissolved in acetone-d6after 0 day (upper) and 3 days (lower). Signals of1looseare indicated by orange triangles. To the suspension was added a CH 2 Cl 2 solution (5 mL) of [Pd( t Bu 2 bpy)(OH 2 ) 2 ](OTf) 2 ·(H 2 O) 2 (9.7 mg, 13.0 µmol, 1.2 equiv. to the dinuclear metallocycle). The reaction mixture was stirred at room temperature for 3 h, and then heated at reflux for 1.5 h. During heating, a colourless solid was precipitated. The resulting precipitate was collected by filtration and dried under reduced pressure. This solid was recrystallised from acetone by vapour diffusion of Et 2 O to afford loosely-twisted 1 loose , [Pd 3 L ( t Bu 2 bpy) 3 ](OTf) 6 ·(H 2 O) 4 , (14.2 mg, 5.21 µmol, 31% in total) as colourless plate crystals. Mp: > 272 °C (decomp.). 1 H NMR (500 MHz, acetone- d 6 , 300 K): δ 8.99 (d, J = 6.0 Hz, 3H), 8.69 (s, 3H), 8.62 (d, J = 1.5 Hz, 3H), 8.47 (d, J = 1.5 Hz, 3H), 8.10 (d, J = 8.0 Hz, 3H), 8.00 (brs, 3H), 7.91 (dd, J = 5.5, 1.0 Hz, 3H), 7.82 (brs, 3H), 7.68 (t, J = 7.5 Hz, 3H), 7.62 (brs, 3H), 7.55 (m, 6H), 7.47 (brs, 3H), 7.19 (d, J = 5.0 Hz, 3H), 6.94 (d, J = 5.0 Hz, 3H), 6.75 (brs, 3H), 4.78 (d, J = 13.0 Hz, 3H), 4.23 (d, J = 13.0 Hz, 3H), 3.21 (d, J = 11.5 Hz, 3H), 1.88 (brs, 3H), 1.54 (s, 27H), 1.43 (s, 27H). 13 C NMR (126 MHz, acetone- d 6 , 300 K): δ 168.6, 166.9, 158.3, 156.4, 151.4, 150.0, 145.6, 141.7, 135.1, 135.1, 134.8, 134.0, 133.8, 133.6, 131.3, 131.3, 127.3, 125.8, 125.7, 123.8, 123.2, 122.8, 120.7, 118.1, 63.1, 60.4, 36.9, 36.7, 30.8, 30.2. 1 H NMR signals of para -phenylene moieties were not fully assigned at 300 K because the rotation of the para -phenylene moieties was so fast that extra cross signals derived from chemical exchange processes appeared in the ROESY spectrum and disturbed the assignment of the signals. So, the 1 H NMR signals of para -phenylene moieties were assigned by 2D 1 H− 1 H COSY and ROESY NMR analyses at 270 K where the rotation of para -phenylene moieties was slow enough. IR (ATR, cm –1 ): 3459 (br), 2975, 1620, 1417, 1240, 1156, 1027, 844. UV-vis (CH 3 CN, 293 K, 82.3 µM): λ max (nm) ( ε (M –1 cm –1 )) = 311 (3.69 × 10 4 ). HRMS (ESI-TOF): m / z = 1100.2410 as [Pd 3 (H –1 L )( t Bu 2 bpy) 3 ](OTf) 4 ] + (calcd 1100.2462). Anal. Calcd for C 102 H 122 F 18 N 12 O 22 Pd 3 S 6 {[Pd 3 L ( t Bu 2 bpy) 3 ](OTf) 6 ·(H 2 O) 4 }: C 45.01, H 4.52, N 6.18; found: C 45.04, H 4.52, N 6.17. 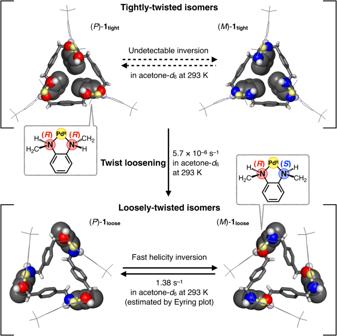Fig. 6: Helicity inversion versus twist loosening of 1tight. Undetectable helicity inversion between (P)- and (M)-1tight, twist loosening from1tightto1looseand fast helicity inversion between (P)- and (M)-1loose. 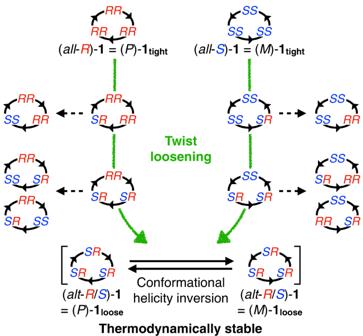Fig. 7: Possible isomers and their isomerisation pathways of 1. All possible diastereomers and their isomerisation pathways for1are shown in this scheme. The black circles indicate the helically twisted macrocyclic structures of1. The notionsRR,SSandSRabove the black circles indicate pairs of the absolute configurations of the amine nitrogen atoms of theortho-phenylenediamine moiety observed in the crystal strictures. The isomerisation pathways to theRSconfiguration are excluded in this scheme, as a pair of the amine nitrogen atoms with theRSconfigurations, with the two amine protons pointing towards the inside of the macrocycle, was not observed experimentally. The green arrows indicate the direct isomerisation pathways from1tightto1loose, and the dotted arrows indicate other possible isomerisation pathways. Crystal data for loosely-twisted Pd 3 L ( t Bu 2 bpy) 3 ·(OTf) 6 ·(C 3 H 6 O) 0.375 ·(H 2 O) 0.5 : C 103.12 H 116.25 F 18 N 12 O 18.88 Pd 3 S 6 , F w = 2679.38, crystal dimensions 0.221 × 0.150 × 0.087 mm 3 , trigonal, space group P -3 c 1, a = 23.8678(5), c = 29.5387(5) Å, V = 14572.9(7) Å 3 , Z = 4, ρ calcd = 1.221 g cm –3 , μ = 44.34 cm –1 , T = 93.15 K, λ (CuK α ) = 1.54178 Å, 2 θ max = 134.130°, 30304/8396 reflections collected/unique ( R int = 0.0431), R 1 = 0.1399 ( I > 2σ( I )), wR 2 = 0.3524 (for all data), GOF = 1.473, largest diff. peak and hole 6.128/–2.917 eÅ –3 . CCDC deposit number 2190129. Asymmetric synthesis of ( M )-enantio-enriched 1 tight from ( S )-3 A CH 2 Cl 2 solution (0.5 mL) of ( S )- 3 (96% ee, 93.5 mg, 513 µmol, 65 equiv.) was added to a CH 2 Cl 2 solution (1.0 mL) of [Pd( t Bu 2 bpy)(OH 2 ) 2 ](OTf) 2 ·(H 2 O) 2 (19.0 mg, 25.5 µmol, 3.2 equiv. ), and this reaction mixture was then cooled to –70 °C. To this solution was added a CH 2 Cl 2 solution (1.0 mL) of L (5.0 mg, 7.93 µmol, 1.0 equiv.) at –70 °C. This reaction mixture was stirred at –70 °C for 4 h. After bringing the reaction mixture to room temperature, Et 2 O was added and the reaction mixture was filtered. The filtrate was evaporated under reduced pressure to afford ( S )-mesityl methyl sulfoxide (87.9 mg, 482 µmol, 94% recovery yield, 95% ee). The precipitate was dissolved in CH 2 Cl 2 and filtered to remove insoluble residue. The filtrate was evaporated and dried in vacuo. After the resulting solid was washed with CHCl 3 , ( M )-enantio-enriched 1 tight was obtained as a pale yellow solid (3.2 mg, 1.19 µmol, 15% yield, 25% ee). The enantiomeric excess was estimated using Δ- 4 as a chiral shift reagent.